Photoswitchable gel assembly based on molecular recognition The formation of effective and precise linkages in bottom-up or top-down processes is important for the development of self-assembled materials. Self-assembly through molecular recognition events is a powerful tool for producing functionalized materials. Photoresponsive molecular recognition systems can permit the creation of photoregulated self-assembled macroscopic objects. Here we demonstrate that macroscopic gel assembly can be highly regulated through photoisomerization of an azobenzene moiety that interacts differently with two host molecules. A photoregulated gel assembly system is developed using polyacrylamide-based hydrogels functionalized with azobenzene (guest) or cyclodextrin (host) moieties. Reversible adhesion and dissociation of the host gel from the guest gel may be controlled by photoirradiation. The differential affinities of α-cyclodextrin or β-cyclodextrin for the trans -azobenzene and cis- azobenzene are employed in the construction of a photoswitchable gel assembly system. Naturally occurring systems build functional assemblies and organs based on a bottom-up strategy through selective molecular recognition by macromolecules, such as DNAs and proteins. Selective molecular recognition among macromolecules is achieved through noncovalent bonds and involves a large number of weak bonding interactions. In recent years, much attention has focused on supramolecular science, the science of noncovalent assembly, in recognition of the importance of specific noncovalent interactions in biological systems and chemical processes. Although many supramolecular architectures have been synthesized [1] , [2] , [3] , [4] , [5] , the self-assembly of macroscopic materials [6] , [7] , [8] , [9] through molecular recognition poses one of the biggest challenges [10] , [11] , [12] . Introduction of a stimulus-responsive guest molecule and its corresponding host molecule to a macroscopic material could provide a means for highly regulated macroscopic assembly through structural changes in the guest moiety triggered by a stimulus. In this way, the interactions between a host and guest can be controllably switched. Here we describe a photoregulated macroscopic gel assembly system using polyacrylamide-based hydrogels functionalized with photoresponsive guest and host molecules. Simple agitation of the photoresponsive guest gel in the presence of the host gel leads to gel adhesion (assembly) through host–guest interactions, and the assembled gels separate into separate pure gels on irradiation with ultraviolet light. The dissociated gels reassemble on visible light irradiation. Placement of a second host gel, which binds the azobenzene (Azo) guest in an alternate conformation favoured by excitation with ultraviolet light, adjacent to the assembly of the first host–guest gels, followed by agitation in water with exposure to ultraviolet light, results in the pairing exchange in the gel assembly, indicating that the gel assembly is photoswitchable. A hydrogel synthesized by copolymerization of monomers bearing host and guest moieties and bis-acrylamide also forms a homogeneous gel assembly and shows the same photoresponsive properties. Preparation of host gels and guest gels α- or β-Cyclodextrin (CD) [13] , [14] , [15] , [16] , [17] , [18] , [19] , [20] and a photoresponsive Azo compound [21] , [22] , [23] , [24] , [25] , [26] , [27] were selected as the host and guest units, respectively. The CD and Azo derivatives were introduced to polyacrylamide-based hydrogels ( Fig. 1 ). All gels were prepared by radical copolymerization under conventional conditions. The gels were cut into 3 or 4 mm pieces using a knife. Host gels were stained with dye, which did not influence the association between the CDs and the guest moieties in the gels, to differentiate the α-CD-gel from the β-CD-gel. The guest gel bearing the Azo-group (Azo-gel) was used without staining, because it was easy to identify on the basis of its orange colour. 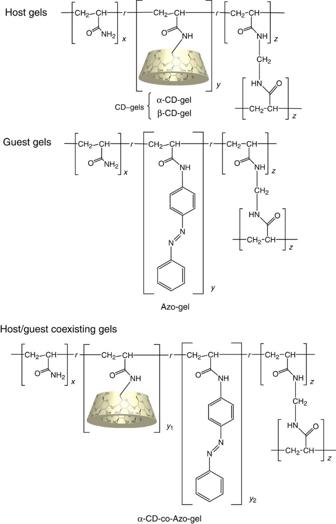Figure 1: Chemical structures of gels. The figure shows the chemical structures of a host gel (α- and β-CD-gels), a guest gel (Azo-gel), and a host/guest coexisting gel (α-CD-co-Azo-gel). The molar ratios of the acrylamide, the host-modified or the guest-modified acrylamide, and theN,N′-methylenebis(acrylamide) are indicated asx,y, andz. Host gels with a mol%x/y/zof 93/5.0/2.0 were used. In this study, guest gels with different Azo group contents (y) were prepared. The characterrin the main chain of the polymers indicates that each monomer was copolymerized randomly. Figure 1: Chemical structures of gels. The figure shows the chemical structures of a host gel (α- and β-CD-gels), a guest gel (Azo-gel), and a host/guest coexisting gel (α-CD- co -Azo-gel). The molar ratios of the acrylamide, the host-modified or the guest-modified acrylamide, and the N,N′ -methylenebis(acrylamide) are indicated as x , y , and z . Host gels with a mol% x / y / z of 93/5.0/2.0 were used. In this study, guest gels with different Azo group contents ( y ) were prepared. The character r in the main chain of the polymers indicates that each monomer was copolymerized randomly. 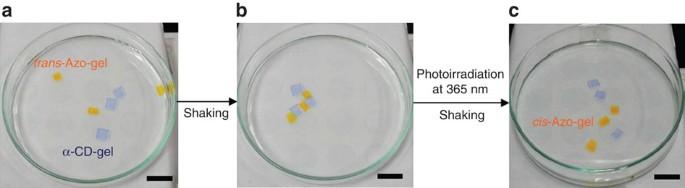Figure 2: Gel assembly and dissociation. Gel assembly of α-CD gel (blue) with thetrans-Azo-gel (orange), and gel dissociation with irradiation with ultraviolet light. (a) Addition of water to the gels in a Petri dish. (b) Agitation of the gels for several minutes led to the assembly of an α-CD-gel/Azo-gel. (c) Photoirradiation at 365 nm led to the dissociation of gels. The scale bar corresponds to 1.0 cm.Supplementary moviesfor the assembly of α-CD-gel withtrans-Azo-gel (Supplementary Movie 1) and the dissociation of the gels after photoirradiation at 365 nm (Supplementary Movie 2) are available.Supplementary Movie 3shows the reference sample for the assembly of the α-CD-gel with the Azo-gel, agitated in water without photoirradiation at 365 nm. Full size image Assembly of the α-CD-gel with the Azo-gel Mixing of the α-CD-gel (blue gel in Figure 2a ) and the Azo-gel with a mol% x / y / z ratio of 97/1.0/2.0 (orange gel), followed by agitation in water, permits adhesion of the α-CD-gel to the Azo-gel to form a combined gel with alternating assembled structures ( Fig. 2b ; Supplementary Movie 1 ). Adhesion of these gels occurred immediately. In control experiments, pieces of a nonfunctionalized blank gel did not stick together or form aggregates with the CD-gels or guest gels. No homogeneous assembly of α-CD-gel/α-CD-gel or Azo-gel/Azo-gel was obtained. These results indicated that α-CD in the host gel bound to the Azo moiety in the guest gel to induce self-assembly of the host and guest gels. Figure 2: Gel assembly and dissociation. Gel assembly of α-CD gel (blue) with the trans- Azo-gel (orange), and gel dissociation with irradiation with ultraviolet light. ( a ) Addition of water to the gels in a Petri dish. ( b ) Agitation of the gels for several minutes led to the assembly of an α-CD-gel/Azo-gel. ( c ) Photoirradiation at 365 nm led to the dissociation of gels. The scale bar corresponds to 1.0 cm. Supplementary movies for the assembly of α-CD-gel with trans- Azo-gel ( Supplementary Movie 1 ) and the dissociation of the gels after photoirradiation at 365 nm ( Supplementary Movie 2 ) are available. Supplementary Movie 3 shows the reference sample for the assembly of the α-CD-gel with the Azo-gel, agitated in water without photoirradiation at 365 nm. Full size image Dissociation of the gels on ultraviolet light irradiation The assembled gels dissociated on light irradiation at 365 nm ( Fig. 2c ; Supplementary Movie 2 ). On irradiation with ultraviolet light, the trans-cis photoisomerization of the Azo units occurred in the Azo-gel. The geometrical structural changes in the Azo unit are thought to trigger dissociation of the host gel/guest gel assembly. To understand the mechanism of gel dissociation on photoirradiation at 365 nm, the interactions between the CDs and the Azo units in the polymers were investigated. A water-soluble copolymer prepared by copolymerization of acrylamide and Azo-acrylamide was mixed with α-CD. A shift in the 1 H-NMR signals assigned to the trans- Azo unit was observed on addition of α-CD, indicating complex formation between the Azo moiety and the α-CD. The estimated association constant ( K a ) for the α-CD/ trans- Azo pair was 2,000 M −1 . After photoirradiation at 365 nm, the 1 H-NMR signals of the cis- Azo units were monitored in the presence and absence of α-CD. The trans / cis Azo ratio was 13/87 on irradiation of light at 365 nm. The K a value for the complexation of α-CD with the cis- form of the Azo group was found to be 35 M −1 . A large difference between the K a values for complexation of α-CD with trans- Azo or cis- Azo was apparent. Adhesion of the gels and dissociation of the assembled gels could be explained as follows. A large number of α-CD molecules bound to the gel could form complexes with the trans- form of the Azo in the guest gel. The adhesion of the α-CD-gel to the Azo-gel is thought to occur through the desired multivalent host–guest interactions. At equilibrium between the α-CD in complex with the Azo moiety and the unbound components, the trans- Azo moiety can alter its geometrical structure to the cis- form on photoirradiation with ultraviolet light outside the binding cavity of the α-CD [28] , [29] . The cis- form weakly interacts with α-CD; however, the affinity of α-CD for the cis- form of Azo is too low to promote gel assembly. As shown in the Supplementary Movie 2 , the cis- Azo-gel could be detached from the α-CD-gel with ease by agitating the gels in water. On the other hand, the trans- Azo-gel remained assembled, even with intense agitation ( Supplementary Movie 3 ). 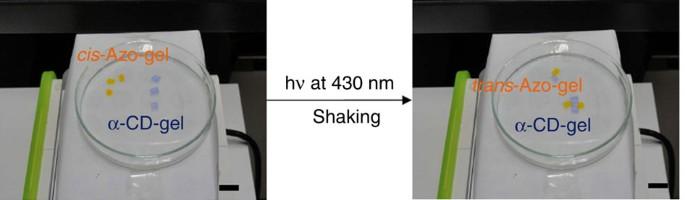Figure 3: Rebinding of the Azo-gel to the α-CD-gel on photoirradiation. Pieces of thecis-Azo-gel prepared with ultraviolet light irradiation and pieces of the α-CD-gel were placed in a Petri dish. These gels were agitated in water with irradiation by visible light at 430 nm. The scale bar indicates 1.0 cm. Reassembly of the host gel with the guest gel The separated α-CD-gels and Azo-gels were found to reassemble on visible light (wavelength at 430 nm) irradiation, as shown in Figure 3 . Binding of the Azo-gels to the α-CD-gels and dissociation of the combined gels were found to be reversible and reproducible. These results indicate that the self-assembly of the macroscopic α-CD- and Azo-gels can be controlled by photoirradiation. We repeated this process and confirmed that the photoswitchable gel assembly could be formed and dissociated at least three times. Figure 3: Rebinding of the Azo-gel to the α-CD-gel on photoirradiation. Pieces of the cis- Azo-gel prepared with ultraviolet light irradiation and pieces of the α-CD-gel were placed in a Petri dish. These gels were agitated in water with irradiation by visible light at 430 nm. The scale bar indicates 1.0 cm. Full size image Photoswitching of the gel-assembly Although the K a value for the complexation of cis -Azo with α-CD is small (35 M −1 ), K a for the complexation with β-CD is 8 times higher (280 M −1 ). β-CD forms a larger host binding cavity than α-CD and tolerantly forms an inclusion complex with both trans- Azo (770 M −1 ) and cis- Azo guest molecules. 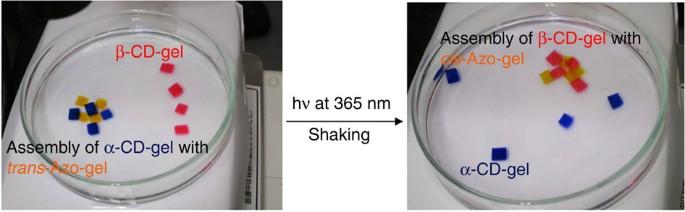Figure 4: Photoswitching of the assembly partner of the Azo-gel. The assembly partner of the Azo-gel switches from the α-CD-gel to the β-CD-gel. Pieces of the β-CD-gel were placed adjacent to the assembly of the α-CD-gel with the Azo-gel. The gel pieces were agitated with exposure to light at 365 nm. When pieces of the β-CD-gel were placed adjacent to the assembly of α-CD-gel with Azo-gel, followed by agitation in water with exposure to light at 365 nm, a pairing exchange reaction occurred, and the Azo-gel/α-CD-gel reassembled to form the Azo-gel/β-CD-gel, as shown in Figure 4 and the Supplementary Movie 4 . Photoisomerization of Azo from trans to cis in the guest gel led to the loss of the adhesion forces with the α-CD-gel. At the same time, photoisomerization induced binding to the β-CD-gel. Table 1 lists the physical properties of the macroscopic self-assemblies between the α- or β-CD-gels and the Azo-gels with different mole contents of the Azo unit. The stress values of the assembly of α-CD-gel/Azo-gel increased with increasing Azo moiety content ( trans- form) in the Azo-gel, 3.5±0.3 kPa at 0.5 mol% and 8.7±0.5 kPa at 1.0 mol%. The adhesion force between the β-CD-gel and the Azo-gel ( cis- form) showed the same trend, that is, the mechanical strength of the assembled gel could be regulated by the mole content of the guest moiety in the guest gel. Figure 4: Photoswitching of the assembly partner of the Azo-gel. The assembly partner of the Azo-gel switches from the α-CD-gel to the β-CD-gel. Pieces of the β-CD-gel were placed adjacent to the assembly of the α-CD-gel with the Azo-gel. The gel pieces were agitated with exposure to light at 365 nm. Full size image Table 1 Physical properties of the macroscopic self-assembled host and guest gels. Full size table Homogeneous gel assembly system As described above, the α-CD-gel adhered to the Azo-gel to provide macroscopic assembly. On irradiation of light at 365 nm, the Azo unit photoisomerized from trans to cis , which led to the dissociation of the assembled gels. Visible light irradiation triggered the reassembly of the host/guest gels. These experimental results clearly showed that the gel assembly system was reversible. Addition of the β-CD-gel to the assembly of the α-CD-gel with the Azo-gel, followed by irradiation with light at 365 nm, induced pair exchange, and the Azo-gel, originally assembled with the α-CD-gel, reassembled with the β-CD-gel in a photoswitchable manner. Introduction of the host and guest molecules into a single gel may yield homogeneous self-assembly of the gels. We examined the assembly of a hydrogel (α-CD- co -Azo-gel) synthesized by copolymerization of the monomers bearing α-CD and the Azo group as pendant groups with acrylamide and bis-acrylamide. 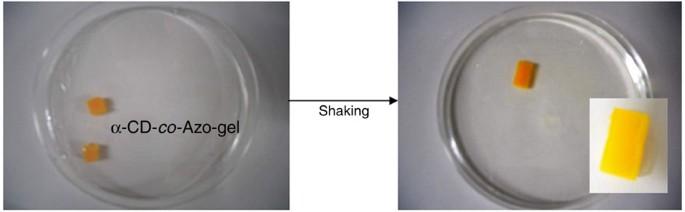Figure 5: Self-assembly of the α-CD-co-Azo-gels. The α-CD-co-Azo-gel was synthesized by copolymerization of acrylamide (x), acrylamido-α-CD (y1), Azo-acrylamide (y2), and bis-acrylamide (z) with a mol%x/y1/y2/zof 81/4/2/13 using AIBN in DMSO at 60 °C. The solvent was replaced with water, and the gel was cut into 5-mm sized pieces using knife. Pieces of the α-CD-co-Azo-gel were shaken in water. As shown in Figure 5 , these gels bound to one another to provide an assembled structure. The stress value of the homogeneous assembly of the α-CD- co - trans -Azo-gels was found to be 6.4±0.2 kPa. The assembled gel was found to dissociate by photoisomerization of Azo from trans to cis . Figure 5: Self-assembly of the α-CD- co -Azo-gels. The α-CD- co -Azo-gel was synthesized by copolymerization of acrylamide ( x ), acrylamido-α-CD ( y 1 ), Azo-acrylamide ( y 2 ), and bis-acrylamide ( z ) with a mol% x / y 1 /y 2 / z of 81/4/2/13 using AIBN in DMSO at 60 °C. The solvent was replaced with water, and the gel was cut into 5-mm sized pieces using knife. Pieces of the α-CD- co -Azo-gel were shaken in water. Full size image An assembly of the Azo-gel with the α-CD-gel separated into separate gels on irradiation at 365 nm, and the gels reassembled on irradiation at 430 nm. The reversible dissociation and adhesion of host/guest gels on the macroscopic scale could be controlled by photoirradiation. A photoswitchable gel assembly system was realized by manipulating the differential binding affinities of the α- and β-CDs towards the trans- / cis- Azo moieties bound to the macroscopic gels. We optimized the fractions of the copolymer components to construct a photoswitchable gel assembly system. Mixing and agitation of the α-CD-gel and β-CD-gel, containing 2.5 mol% of the CD unit, along with the trans- Azo-gel containing 1.5 mol% of the Azo unit, resulted in the selective adherence of the α-CD-gel to the trans- Azo-gel, as shown in the Supplementary Movie 5 . The higher affinity of the trans- Azo-gel for the α-CD-gel ( K a(α−CD− trans− Azo) =2,000 M −1 ) than for the β-CD-gel ( K a(β−CD− trans− Azo) =770 M −1 ) led to the selective binding of the α-CD-gel to the trans- Azo-gel in water. Exposure of a composite material of the α-CD-gel and trans- Azo-gel to 365 nm light resulted in dissociation, and the resultant cis- Azo-gel formed an assembly with the β-CD-gel. The assembly of the α-CD-gel with the trans- Azo-gel switched completely to the assembly of the β-CD-gel with the cis- Azo-gel on light irradiation at 365 nm. The trans- Azo-gel, which was obtained by photoisomerization of the cis- Azo-gel on light irradiation at 430 nm in the presence of the β-CD-gel, readhered to the α-CD-gel with agitation at high speeds. The affinity of the α-CD-gel towards the trans- Azo-gel is strong enough to support a bound state, even with violent agitation in water. Increasing the concentration of the trans- Azo group in the Azo-gel from 0.5 to 1.0 mol% increased the stress values for the assembly with the α-CD-gel. The same trend was observed for the assembly of the cis- Azo-gel with the β-CD-gel. These results indicated that the number of host and guest molecules on the surface of the gels was important in the gel assembly system. We found that the mechanical strength of the host/guest gel assembly was proportional to the contacting surface area of the gels. The surface density of the host and guest moieties is expected to govern the mechanical strength of the assembled gel. The mechanical strength of the assembled gel could be regulated by changing the mole content of the host or guest moiety in the gels. Mixing of 2 mol% bis-acrylamide with 92 mol% acrylamide, 4 mol% acrylamido-α-CD, and 2 mol% Azo-acrylamide in dimethylsulfoxide (DMSO), resulted in copolymerization and gelation in the presence of 2,2′-azobis(isobutyronitrile) (AIB). The gel would dramatically shrink if the DMSO were changed with water. Gel shrinkage indicated the formation of host–guest complexes within the gel in the presence of water. A stable α-CD- co -Azo-gel was obtained by changing the mole content of the bis-acrylamide from 2 to 13. An α-CD- co -Azo-gel bearing both host and guest molecules in the same gel also yielded assembly. All systems in this study exhibited excellent photoresponsive properties in gel assemblies. We anticipate that the photoswitchable self-assembly demonstrated in this study can be applied to the production of a variety of functionalized materials on the macroscopic scale. Materials Acrylamido-α-CD and acrylamido-β-CD were prepared according to the procedures previously reported by our group [11] . CD-gels were prepared by copolymerization of acrylamide (6.2 mmol), 6-acrylamido-CD (CD=α- or β-CD, 0.33 mmol) and N,N′ -methylenebis(acrylamide) (0.12 mmol) by radical polymerization initiated by the redox pair ammonium peroxodisulfate and N,N,N′,N′- tetramethylethelenediamine in water. A guest gel containing the azobenzene group (Azo-gel) was prepared by copolymerization of acrylamide, an acrylamide derivative bearing an Azo moiety, and N,N′ ‐methylenebis(acrylamide) by radical polymerization using AIBN in DMSO at 60 °C. 1 H-NMR spectra of the Azo-monomer in CDCl 3 and the Azo-polymer before and after irradiation of ultraviolet light and visible light in D 2 O are shown in the Supplementary Figures S1-S3 , respectively. An acrylamide gel bearing neither CDs nor guest moieties was also prepared as a blank gel in a similar manner. A hydrogel bearing both α-CD and the Azo group was synthesized by copolymerization of acrylamido-α-CD, Azo-acrylamide, and bis-acrylamide using AIBN in DMSO at 60 °C. A water-soluble guest polymer bearing an Azo moiety was prepared by copolymerization of acrylamide and Azo-acrylamide by a radical polymerization using AIBN in DMSO at 60 °C. These soluble guest polymers, bearing an Azo group in their side chains, were used for the 1 H-NMR measurements to determine the association constants ( K a ) for the complexation of CDs with these guests and the ratio of the trans- and cis- isomers of the Azo moiety. Pieces of the CD-gels were stained by soaking these gels in the solutions of the dyes: α-CD-gel (blue, FD&C Blue No. 1 (brilliant blue FCF)) and β-CD-gel (red, FD & C Red No.3 (erythrosine)). Guest gels containing Azo were used without straining. Azo-acrylamide p- Aminoazobenzene (5.0 g, 25 mmol) and triethylamine (4.0 ml, 29 mmol) were dissolved in 180 ml dried THF on an ice bath. Acryloyl chloride (2.3 ml, 29 mmol) was added to the solution of p- aminoazobenzene. The solution was stirred for 3.5 h on an ice bath. The precipitate was removed by filtration, and the filtrate was concentrated under reduced pressure. The obtained crude product was purified by recrystallization from CH 2 Cl 2 (2.5 g, 40%). 1 H-NMR (500 MHz, CDCl 3 ): δ 7.62 (d, 2H, J =9.0 Hz), 7.89 (d, 2H, J =9.0 Hz), 7.75 (d, 2H, J =9.0 Hz), 7.50 (dd, 1H, J =9.0, 9.0 Hz), 7.46 (d, 2H, J =9.0 Hz), 7.36 (brs, 1H), 6.48 (d, 1H, J =17.0 Hz), 6.27 (dd, 1H, J =10.0, 17.0 Hz), 5.82 (d, 1H, J =10.0 Hz). ESI-MS m / z 252 [M+1] + , 274 [M+Na] + . A water-soluble Azo-polymer The Azo-polymer was prepared by radical polymerization in DMSO at 60 °C for 48 h, using AIBN as the initiator (monomer concentration=4.2 M). The ratio of acrylamide (0.27 g, 3.9 mmol) and Azo-acrylamide (10 mg, 40 μmol) was 99:1. The molar ratio of the monomer to the AIBN (3 mg, 20 μmol) was 100:0.5. Argon was bubbled through the solution for 30 min before heating. After 48 h, the product was purified three times by precipitation in MeOH, followed by drying under vacuum. An orange solid (0.24 g) was obtained. 1 H-NMR (500 MHz, D 2 O): δ 7.1–7.5 (m, broad, 9H, aromatic protons), 0.9–2.0 (broad, principal chain protons). α-CD- co -Azo-gel α-CD- co -Azo-gel was prepared by copolymerization of acrylamide (6.2 mmol), acrylamido-α-CD (0.31 mmol), Azo-acrylamide (0.12 mmol), and N, N′ -methylenebis(acrylamide) (0.97 mmol) using AIBN (0.20 mmol) in 5.0 ml of DMSO at 60 °C. The gel was purified by washing with large amounts of DMSO, followed by exposure to water over several hours, then repeated washing with water. Measurements 1 H-NMR spectra were recorded at 500 MHz with a JEOL ECA-500 NMR spectrometer. Chemical shifts were referenced to the solvent values ( δ 2.49 p.p.m. for DMSO, δ 4.79 p.p.m. for HOD, and δ 7.25 p.p.m. for CDCl 3 ). Infrared spectra were recorded with a JASCO FT-IR-410 spectrometer. The mechanical properties of the gel-assemblies were measured using a mechanical tension testing system (Rheoner, RE-33005, Yamaden). The host gel and guest gel were pushed together to contact one another. The stress of 1×1 cm length samples was measured at a speed of 0.1 mm per sec at room temperature. Macroscopic self-assembly between the host gels and guest gels was performed in water. Each gel was placed in a Petri dish; 30 ml water was added; and the dish was agitated (EYELA CM-1000) for a few minutes at room temperature. Photoisomerization of the Azo groups in the Azo-gel was carried out using a 300-W Xe lamp (Asahi Spectra MAX-301) equipped with a band-pass filter (LX0365) for ultraviolet light and a band-pass filter (MX0430) for visible light. Determination of the apparent association constants The interactions of the CDs with the trans- or cis- Azo groups in the Azo-polymer were monitored by 1 H-NMR. The 1 H-NMR spectral changes of trans - or cis- Azo moieties in the Azo-polymer on addition of α-CD or β-CD are shown in the Supplementary Figures S4-S7 , respectively. The apparent association constants ( K a ) of CDs with guest moieties in the soluble guest polymers were estimated using Benesi–Hildebrand plots of 1/Δδ obs versus 1/C CD , as shown in the Supplementary Figure S8 . The K a values include errors within ±10%. How to cite this article: Yamaguchi, H. et al . Photoswitchable gel assembly based on molecular recognition. Nat. Commun. 3:603 doi: 10.1038/ncomms1617 (2012).